Bound vortex dipoles generated at pinning centres by Meissner current One of the phenomena that make superconductors unique materials is the Meissner-Ochsenfeld effect. This effect results in a state in which an applied magnetic field is expelled from the bulk of the material because of the circulation near its surface of resistance-free currents, also known as Meissner currents. Notwithstanding the intense research on the Meissner state, local fields due to the interaction of Meissner currents with pinning centres have not received much attention. Here we report that the Meissner currents, when flowing through an area containing a pinning centre, generate in its vicinity two opposite sense current half-loops producing a bound vortex–antivortex pair, which eventually may transform into a fully developed vortex–antivortex pair ultimately separated in space. The generation of such vortex dipoles by Meissner currents is not restricted to superconductors; similar topological excitations may be present in other systems with Meissner-like phases. In the framework of the standard model [1] for describing fundamental particles and their interactions, all sub-atomic particles have an associated twin: an antiparticle. These twins are identical except, for example, for their opposite charge or helicity, and the laws of nature are very nearly symmetrical for a particle and its antiparticle [2] . However, as a general rule, particle–antiparticle pairs can coexist only in a metastable state as they tend to annihilate each other. The universal duality is reflected in the vortex physics of superconductors and superfluids, where vortex–antivortex (v-av) pairs can be induced by different causes: by undergoing a Kosterlitz-Thouless transition [3] , which can result, for example, in the formation of self-ordered vortex–antivortex states in ultracold Fermi gases [4] or polariton condensates [5] , through photon absorption [6] , [7] , [8] or thermal activation [9] ; by a confinement potential with an appropriate symmetry in superconducting samples [10] , [11] and Bose–Einstein condensates [12] ; by an inhomogeneous magnetic field, such as one resulting from dipolar magnetic nanostructures in the vicinity of the superconductor [13] , [14] or by a moving obstacle potential that generates a Karman v-av street in classical gases and polariton quantum fluids [15] , [16] , [17] . Vortex matter in superconductors has been extensively studied in the mixed state [18] . Unluckily, the same vortices that stabilize superconductivity in high magnetic fields, compromise its key characteristic, its ability of carrying electrical current with zero resistance. Unpinned vortices move in response to an applied electrical current, thus dissipating energy and destroying the zero-resistance state [19] , [20] . As a result, introducing pinning centres, which efficiently immobilize vortices in the mixed state, became a problem that has plagued scientists trying to engineer real-world applications of superconductors for decades [21] , [22] , [23] , [24] . However, almost no attention has been paid to the role of pinning centres in the behaviour of superconductors in the Meissner state. Here, we report on direct experimental detection of v-av pairs bound to pinning centres situated close to the superconductor edge, where Meissner currents flow. We have used high-resolution low-temperature scanning Hall probe microscopy to visualize this novel bound vortex dipole state. By scanning various areas of the sample with pinning centres, we have found excellent correspondence between the observed orientations of the vortex dipoles and the direction of the Meissner screening current. Our experimental finding is supported by theoretical modelling in the framework of the time-dependent Ginzburg-Landau (TDGL) equations. To the best of our knowledge, these new bound vortex dipoles are qualitatively different from previously studied v-av pairs in superconductors. We found that the magnetic flux carried by each pole of the vortex dipole is not quantized, but it is proportional to the Meissner current density. Determination of pinning sites Our experiments have been carried out on a 200-nm-thick superconducting Pb film with randomly distributed pinning centres. There exist several methods to introduce pinning centres in superconductors, such as lithographically made well-controlled pinning sites [25] , [26] , ion-irradiation-introduced point defects [27] , grain boundaries [28] , thickness variations [29] and so on. Most of these methods lead to the suppression of the superconducting order parameter at the pinning sites that makes them energetically favourable for vortices to localize on [30] . In our sample, the pinning sites are created unintentionally during sample preparation. To identify the pinning centres, we have performed a series of field-cooling experiments. As shown in Fig. 1a,b , during field-cooling, vortices prefer to be trapped at positions where pinning sites are located. With increasing cooling fields, more and more pinning sites are occupied by single quantum vortices (Φ 0 -vortices, where Φ 0 = h /2 e with h the Planck constant and e the electron charge). After all the pinning sites are occupied by Φ 0 vortices, multiquanta vortices and interstitial vortices (vortices sitting in between pinning sites) start to appear ( Fig. 1c ). At B 0 =2.4 G ( Fig. 1d ), eight multiquanta vortices could be observed in the scanned area, suggesting the presence of relatively strong pinning centres at their positions. We define the vortices located at these sites as pinned vortices (see, for example, the dashed circle in Fig. 1c ) and the other vortices as interstitial (see, for example, the dotted circle in Fig. 1c ). We found that a maximum of three flux quanta can be trapped by the pinning centres at magnetic fields up to 11 G ( Fig. 1h ). This is similar to a superconductor with antidots as pinning centres, where multiquanta vortices are formed and the interaction between pinning centre and vortices becomes purely repulsive only when a saturation number n s is reached [31] , [32] , [33] , [34] . 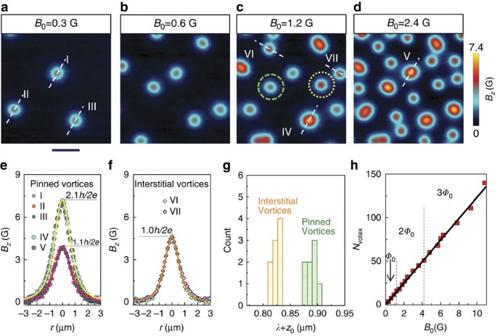Figure 1: Distribution of vortices after field cooling toT=4.2 K reveals the distribution of pinning centres. (a–d) Scanning Hall probe microscopy images taken at the applied magnetic fieldB0=0.3 G (a), 0.6 G (b), 1.2 G (c) and 2.4 G (d). Scale bar, 4μm. At the lowest fields (a,b), only single quantum vortices are observed which are located at pinning centres. At higher fields (c,d), when all the pinning centres are occupied (c), giant vortices with vorticityL=2 and interstitial single quantum vortices appear. Interstitial vortices (like that indicated by the dotted circle inc) appear brighter than pinned vortices (indicated by the dashed circle). The field profiles, measured along the dashed lines I to VII inaandc, are shown ineandffor pinned and interstitial vortices, respectively. Hereris the distance from the centre of a vortex. The solid lines ineandfare fittings based on the monopole model. Since at pinning sites the local density of superconducting charge carriers is reduced and hence the penetration lengthλis larger than outside these sites, the magnetic field induced by a pinned vortex spreads over a wider area and the field magnitude at the vortex centre appears lower as compared with those for an interstitial vortex. The histograms ofλ+z0values calculated from the monopole model (g) yield an average value of 0.89 and 0.82 μm for the pinned and interstitial vortices, respectively, showing that indeed, interstitial vortices correspond to a smallerλas compared with pinned ones. (h) Total vorticity of vortices observed in the scanned area as a function of applied field. The solid line is the expected valueNvortex=B0S/Φ0, whereS=16 × 16 μm2is the size of scanned area and Φ0=h/2eis flux quantum. The vertical dashed lines indicate the fields above which 2Φ0- and 3Φ0-vortices appear. Figure 1: Distribution of vortices after field cooling to T =4.2 K reveals the distribution of pinning centres. ( a – d ) Scanning Hall probe microscopy images taken at the applied magnetic field B 0 =0.3 G ( a ), 0.6 G ( b ), 1.2 G ( c ) and 2.4 G ( d ). Scale bar, 4μm. At the lowest fields ( a , b ), only single quantum vortices are observed which are located at pinning centres. At higher fields ( c , d ), when all the pinning centres are occupied ( c ), giant vortices with vorticity L =2 and interstitial single quantum vortices appear. Interstitial vortices (like that indicated by the dotted circle in c ) appear brighter than pinned vortices (indicated by the dashed circle). The field profiles, measured along the dashed lines I to VII in a and c , are shown in e and f for pinned and interstitial vortices, respectively. Here r is the distance from the centre of a vortex. The solid lines in e and f are fittings based on the monopole model. Since at pinning sites the local density of superconducting charge carriers is reduced and hence the penetration length λ is larger than outside these sites, the magnetic field induced by a pinned vortex spreads over a wider area and the field magnitude at the vortex centre appears lower as compared with those for an interstitial vortex. The histograms of λ + z 0 values calculated from the monopole model ( g ) yield an average value of 0.89 and 0.82 μm for the pinned and interstitial vortices, respectively, showing that indeed, interstitial vortices correspond to a smaller λ as compared with pinned ones. ( h ) Total vorticity of vortices observed in the scanned area as a function of applied field. The solid line is the expected value N vortex = B 0 S /Φ 0 , where S =16 × 16 μm 2 is the size of scanned area and Φ 0 = h /2 e is flux quantum. The vertical dashed lines indicate the fields above which 2Φ 0 - and 3Φ 0 -vortices appear. Full size image To quantify the magnetic flux carried by the vortices, we used the monopole model (see Methods) to fit the magnetic profiles as indicated by the solid lines in the scanning Hall probe microscope (SHPM) images [35] . The fitting provides the carried magnetic flux Φ and the value of λ + z 0 , where λ is the penetration depth and z 0 is the distance between the sample surface and the two-dimensional electron gas (2DEG) of the Hall cross. Notice that z 0 is a constant in the used lift-off scanning mode [35] . The main source of error when using the monopole model to fit the vortex profiles comes from the overlap of the stray magnetic fields of the adjacent vortices. For pinned vortices ( Fig. 1e ), the fitting yields Φ=(1.1±0.15) h /2 e for the vortices I, II, III, and Φ=(2.1±0.15) h /2 e for the vortices IV, V, whereas for the interstitial vortices VI and VII ( Fig. 1f ), Φ=(1.0±0.15) h /2 e . We notice from the field profiles that the magnetic field at the centre of interstitial vortices is higher than that of pinned vortices. This is also reflected by the shading of the colour from bright red for interstitial vortices to reddish brown for pinned ones in Fig. 1c . To further elucidate this difference, we show in Fig. 1g the histogram of the λ + z 0 values for the observed single quantum vortices. The histogram demonstrates a separation of λ + z 0 into two groups, with an average value of 0.89 μm for pinned vortices and 0.82 μm for interstitial vortices. Given that z 0 is constant, this indicates that the magnetic field of the vortices sitting on pinning sites spreads over a larger area, corresponding to a larger local value of λ . This enlargement of λ implies that the related superfluid density, ρ s ( T ) ∝ 1/λ 2 ( T ) (ref. 36 ), at the pinning centres is reduced as compared with the rest of the superconducting area. Besides the quantification of the magnetic flux, the images also reveal shape differences between the vortices. Although the local magnetic field distributions labelled as IV and V are nearly circular, some other multiquanta patterns clearly exhibit an elongated shape. As all the pinning sites are naturally generated, one reason for such an elongation might be the asymmetry of the pinning potential, which leads to a deformation of a multiquanta vortex. Alternatively, these elongated field patterns can correspond to relatively large pinning centres where vortex clusters, rather than multiquanta vortices, tend to form (see also the simulation results in Fig. 4 ). Figure 4: Simulation results. ( a ) Variations of mean free path l in a 20 × 20 μm 2 superconductor with six pinning sites. 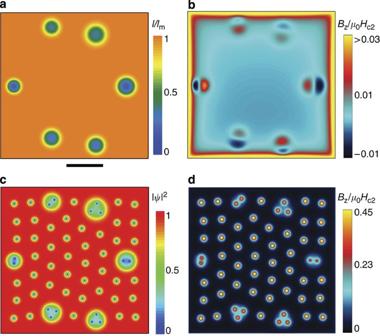Figure 4: Simulation results. (a) Variations of mean free pathlin a 20 × 20 μm2superconductor with six pinning sites. Scale bar, 5μm. (b) Magnetic field in the superconductor after performing zero-field cooling followed by an increase of the applied field toB0=0.05μ0Hc2. At all the six pinning sites, vortex dipoles appear due to distortions of the Meissner current flowing along the borders. (c,d) The distribution of squared order parameter and the magnetic field, respectively, in the superconductor cooled atB0=0.05μ0Hc2. Vortex clusters are formed at the defined pinning sites. Scale bar, 5μm. ( b ) Magnetic field in the superconductor after performing zero-field cooling followed by an increase of the applied field to B 0 =0.05 μ 0 H c2 . At all the six pinning sites, vortex dipoles appear due to distortions of the Meissner current flowing along the borders. ( c , d ) The distribution of squared order parameter and the magnetic field, respectively, in the superconductor cooled at B 0 =0.05 μ 0 H c2 . Vortex clusters are formed at the defined pinning sites. Full size image Visualization of vortex dipoles Having detected the locations with strong pinning, now we can analyse the effect of pinning centres on the Meissner supercurrents, which is the main result of this paper. To perform this, we start with zero-field cooling down to a temperature below the critical temperature T c and subsequently we slowly increase the external field while at the same time mapping the field distribution near the superconductor surface. As seen from Fig. 2a–f , several vortex dipoles, corresponding to bound vortex–antivortex pairs with opposite magnetic field direction, appear and their field increases with the increase of the external magnetic field. The field profiles of the vortex dipoles, measured along the dashed lines in Fig. 2a, c and f and shown in Fig. 2g , clearly reveal an antisymmetric shape, which is somewhat masked in the SHPM images by the colour scale. We notice that the centres of the dipoles overlap precisely with the pinning sites, defined from the established positions of giant vortices in Fig. 1d and indicated with the yellow circles in Fig. 2f . The observed vortex dipoles have nearly the same in-plane orientation in a 16 × 16 μm 2 scanned area (see also Fig. 3a ) and they only appear in the superconducting state. This rules out phase separation or the presence of ferromagnetic impurities in our sample. 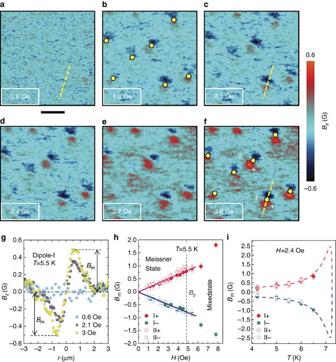Moreover, no ferromagnetic impurities were intentionally introduced in our samples during the preparation process. Figure 2: Vortex dipoles observed at pinning centres. (a–f) Scanning Hall probe microscopy images taken after first performing zero-field cooling to 5.5 K and then increasing external field to 0.6 G (a), 1.8 G (b), 2.1 G (c), 2.4 G (d), 2.7 G (e), 3 G (f). Scale bar, 4μm. The yellow circles inbandfindicate the locations where the giant vortices appear in the field cooling image shown inFig. 1d. As the external magnetic field is increased, vortex dipoles with nearly the same orientation appear at these locations. (g) Magnetic field profiles of a vortex dipole, which are measured along the dashed line ina,candf. (h) Magnetic fieldBmat the centres of bound vortices and antivortices in the dipoles, labelled by I and II inf, as a function of the applied field atT=5.5 K. Below the penetration fieldBp=4.8 G, the measured values ofBm(B0) are well fitted by linear functions. AboveBp, due to the penetration of vortices from the edge, this linear dependence is violated. (i) Magnetic field at the centre of vortex and antivortex forming dipoles I and II as a function of temperature atB0=2.4 G. The dashed lines are fit with equation (1). The data, in agreement with the equation, confirm that an increase ofλ, resulting from a temperature rise, enhances the local current densityJnear the pinning sites. The error bars inhandimainly come from the noise in the data and the error in the background determination, and represent standard errors. Figure 2: Vortex dipoles observed at pinning centres. ( a – f ) Scanning Hall probe microscopy images taken after first performing zero-field cooling to 5.5 K and then increasing external field to 0.6 G ( a ), 1.8 G ( b ), 2.1 G ( c ), 2.4 G ( d ), 2.7 G ( e ), 3 G ( f ). Scale bar, 4μm. The yellow circles in b and f indicate the locations where the giant vortices appear in the field cooling image shown in Fig. 1d . As the external magnetic field is increased, vortex dipoles with nearly the same orientation appear at these locations. ( g ) Magnetic field profiles of a vortex dipole, which are measured along the dashed line in a , c and f . ( h ) Magnetic field B m at the centres of bound vortices and antivortices in the dipoles, labelled by I and II in f , as a function of the applied field at T =5.5 K. Below the penetration field B p =4.8 G, the measured values of B m ( B 0 ) are well fitted by linear functions. Above B p , due to the penetration of vortices from the edge, this linear dependence is violated. ( i ) Magnetic field at the centre of vortex and antivortex forming dipoles I and II as a function of temperature at B 0 =2.4 G. The dashed lines are fit with equation (1). The data, in agreement with the equation, confirm that an increase of λ , resulting from a temperature rise, enhances the local current density J near the pinning sites. 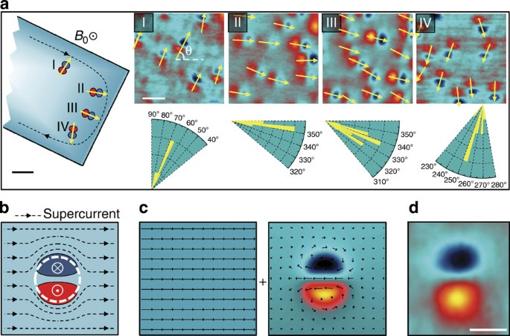The error bars in h and i mainly come from the noise in the data and the error in the background determination, and represent standard errors. Figure 3: Mechanism of the vortex dipole formation. (a) Scanning Hall probe microscopy images (I–IV) taken at different locations of the sample as schematically indicated in the left panel. The arrows highlight the direction of the dipoles. Red and blue colours correspond to magnetic field pointing outward and inward, respectively. As follows from the histograms of dipole direction, which are shown below images I to IV, within one and the same scanned location all the dipoles have similar orientations. Scale bar, 100μm; inset, 4μm. (b) Schematic view of a supercurrent flowing through the area around a pinning centre, which is shown by the dashed circle. The clockwise and counterclockwise current flows result in the formation of a vortex dipole. The current distribution inbis equivalent to a uniform current flow (c) superimposed with two current loops with opposite polarities (c). The arrows incindicate the current density vector distributions, while the colour maps represent the magnetic fieldBz, induced by the corresponding currents. The simulated dipole demonstrates a very good qualitative resemblance with experimentally observed vortex dipole shown ind. Scale bar, 2μm. Full size image Figure 3: Mechanism of the vortex dipole formation. ( a ) Scanning Hall probe microscopy images (I–IV) taken at different locations of the sample as schematically indicated in the left panel. The arrows highlight the direction of the dipoles. Red and blue colours correspond to magnetic field pointing outward and inward, respectively. As follows from the histograms of dipole direction, which are shown below images I to IV, within one and the same scanned location all the dipoles have similar orientations. Scale bar, 100μm; inset, 4μm. ( b ) Schematic view of a supercurrent flowing through the area around a pinning centre, which is shown by the dashed circle. The clockwise and counterclockwise current flows result in the formation of a vortex dipole. The current distribution in b is equivalent to a uniform current flow ( c ) superimposed with two current loops with opposite polarities ( c ). The arrows in c indicate the current density vector distributions, while the colour maps represent the magnetic field B z , induced by the corresponding currents. The simulated dipole demonstrates a very good qualitative resemblance with experimentally observed vortex dipole shown in d . Scale bar, 2μm. Full size image To further understand the nature of this bound vortex–antivortex pairs, we have studied their magnetic-field and temperature dependencies. Figure 2h displays B m , the amplitude of the field profile for vortices and antivortices forming a vortex dipole, as a function of the external magnetic field. Clearly, the field amplitude B m follows a linear dependence on B 0 in the Meissner state, whereas at the vortex penetration field B p the dependence starts to deviate from linearity. We have also characterized the vortex dipoles at various temperatures for a fixed external field. The temperature dependence of the amplitude B m for the vortices (antivortices), forming dipoles I and II in Fig. 3f , is presented in Fig. 2i by the filled and open diamonds (squares), showing an increase of B m as the temperature rises. We find an explanation of these phenomena in the nature of Meissner currents. For superconductors, when the external field is lower than the penetration field B p =(1− N ) μ 0 H c1 , where N is the demagnetization factor due to the sample geometry and μ 0 H c1 is the lower critical field, a Meissner current, proportional to the external field, will be induced that flows along the sample borders. According to the London theory, in the vicinity of the superconductor boundary, the penetrated magnetic field decays exponentially over a characteristic length λ , B ( r )= B 0 exp(− r /λ), where λ is the penetration depth, r is the distance from the boundary and B 0 is the external field [36] . In the two-fluid model [37] , the temperature dependence of λ takes the expression with λ(0) the penetration depth at zero temperature. By using the Maxwell equations, the corresponding Meissner current density is Accordingly, the data presented in Fig. 2h behave linearly with B 0 until B p is reached, where a deviation from the linear dependence is observed due to the penetration of flux inside the sample. Similarly, the experimental data in Fig. 2i can be well fitted by introducing a conversion constant C between the current and the magnetic field amplitude of the v-av forming the dipole, B m ( r , T )= CJ ( r , T ), as shown by the dashed lines. As implied by equation (1), if the penetration depth is significantly smaller than the distance r between a pinning site and the nearest border of the sample, the dependence of the Meissner current density J on λ is dominated by the exponential function exp(− r /λ). This means that an increase of λ , resulting from a temperature rise, enhances the local current density J near the pinning site. Therefore, in the corresponding temperature range, the magnetic field B m increases with temperature. In contrast to that, in the situation where λ becomes appreciably larger than r , the current density J can be approximated by B 0 / λ , so that the Meissner current and the dipole magnetization vanish at T = T c . However, as r is much larger than λ (0) for the pinning sites under consideration, the inequality λ ( T )> r can be obeyed only for temperatures very close to T c , which fall outside of our experimental capabilities. Mechanism of the vortex dipole formation The presented experimental data suggest that the vortex dipoles are indeed strongly related to pinning and to the Meissner current. As the Meissner screening current, which flows along the sample border, changes direction at the corners, it is expected that the vortex dipole orientation follows the same trend. We mapped the dipole orientation at a few selected locations as shown in Fig. 3a . As indicated by the arrows, the vortex dipole axes are approximately perpendicular to the expected direction of the Meissner current in the scanned area. In the histogram below each of the images show a clear preferential direction of the vortex dipoles. Nevertheless, some deviations are seen. We argue that these deviations from the preferential direction can arise from local distortions of the Meissner current, which are caused by neighbouring pinning centres. As follows from Fig. 1g , the penetration depth at pinning sites is considerably larger, thus corresponding to smaller superconducting carrier density. When a supercurrent flows through an area with a pinning site, the current tends to follow a path with higher superconducting carrier density, as schematically shown in Fig. 3b . The resulting current density distribution can be represented as a superposition of a uniform current flow, which does not contribute to the magnetic field B z , and two current loops with opposite polarity, as shown in Fig. 3c . The simulated magnetic field generated by current loops is also displayed in Fig. 3c . The shown field pattern agrees fairly well with the experiment ( Fig. 3d ). This model also explains the dependence of the magnetic fields, induced by the observed vortex dipoles, on the Meissner current strength. Of course, for a particular vortex dipole, the field pattern is affected also by the geometric and material parameters, which characterize the corresponding pinning centre. Simulations To further elucidate the described mechanism of the vortex dipole formation, we performed detailed simulations using the TDGL equations. In our calculations, we consider a superconducting film with a thickness of 200 nm and with lateral sizes X × Y =20 × 20 μm 2 . The pinning centres are introduced as well-defined areas with reduced local values of the mean free path l . As shown in Fig. 4a , six pinning centres are located in the vicinity of the sample borders. The TDGL simulations, corresponding to zero-field cooling followed by an increase of the applied magnetic field, reveal a magnetic field pattern with six vortex dipoles at the pinning sites (see Fig. 4b ). In line with the experimental observations, the dipole axes are perpendicular to the direction of the Meissner current and the magnitude of the magnetic fields, induced by a dipole, decreases with increasing distance between the corresponding pinning centre and the nearest border of the sample. Of course, this magnitude depends also on the lateral size and depth of the pinning potential, which are determined by the spatial variations of the ratio l / l m . Figure 4c,d shows the calculated distributions of the squared order parameter and magnetic field, respectively, which correspond to field cooling. Similar to the results shown in Fig. 1 , vortices tend to stay at the pinning sites. However, for the used set of parameters, pinned vortices form vortex clusters rather than giant vortices. This resembles the effect observed in superconducting films with blind antidots [29] , where, due to the large size of blind holes, a trapped n Φ 0 multiquanta vortex at the antidot explodes into n individual Φ 0 vortices in the bottom superconducting layer. In our experiment, owing to the limited space resolution, vortex dimers or clusters cannot be resolved. However, we do observe that some multiquanta vortices clearly exhibit an elongated shape as shown in Fig. 1d . We have presented direct experimental evidence of bound vortex–antivortex pairs, named vortex dipoles, appearing in the Meissner state of a superconductor. We show that these vortex dipoles nucleate as a result of the interaction between pinning sites and the flowing Meissner supercurrent. We have observed the nucleation of these bound pairs and studied their evolution as a function of the magnetic field and temperature, revealing that the vortex dipoles are qualitatively different from the vortex–antivortex pairs usually observed in the mixed state of a type-II superconductor. In particular, the magnetic flux corresponding to either pole of a vortex dipole is not quantized and its value is determined by the local density of the flowing Meissner currents (and hence by the strength of the external magnetic field) and by the variation of the superconducting parameters at the pinning site and its geometry. At the same time, our theoretical calculations show that, depending on the size and shape of a pinning centre, vortex dipoles may evolve into fully developed vortex–antivortex pairs, ultimately separated in space, if the current density flowing nearby the pinning site is high enough (see Supplementary Fig. 1 ). However, the corresponding current densities significantly exceed the Meissner current densities achievable at the pinning centres in our experimental sample. In view of this, our bound vortex dipoles may be classified as precursors of fully developed vortex–antivortex, in which a vortex (antivortex) carries just one flux quantum. On the one hand, our findings prove a way to detect hidden submicron defects in superconducting materials in a non-invasive way, which is rather difficult by using a conventional X-ray method. On the other hand, our findings reveal the fundamental importance of studying the effect of pinning sites in the Meissner state of superconductors. In addition, tuning the size and/or symmetry of the pinning sites may result in new facets of this phenomenon, for instance in a superconductor with periodic artificial antidots. Moreover, the relevance of the observed vortex dipoles is not restricted to superconductors, but it is of importance for further analysis of similar topological excitations in superfluids and Bose–Einstein condensates, which also present a Meissner-like phase, such as 4 He atoms flowing in a superfluid [38] and chiral edge currents in bosonic ladders [39] . Experimental setup The Pb film was prepared on a Si/SiO 2 substrate using an ultrahigh vacuum (3 × 10 −8 Torr) electron beam evaporator calibrated with a quartz monitor. The substrate was cooled to 77 K by liquid nitrogen to ensure the homogeneous growth of Pb. On top of Pb, a 5-nm-thick Ge layer is deposited to protect the sample surface from oxidation. The starting materials were 99.999% pure Pb and 99.9999% pure Ge. The surface is investigated by atomic force microscopy (AFM) and a roughness of 0.16 nm is found (see Supplementary Fig. 2 ). The critical temperature T c =7.25 K is determined using local ac susceptibility measurements ( Supplementary Fig. 3 ). The local magnetic field distribution was mapped using a low-temperature SHPM from Nanomagnetics Instruments, with a temperature stability better than 1 mK and magnetic field resolution of 0.1 G. All the images are recorded in the lift-off mode by moving the Hall cross above the sample surface at a height of ~0.6 μm. In all the measurements, the magnetic field is applied perpendicularly to the sample surface. Monopole model In the limit of ( r 2 + z 0 ) ≫ λ 2 , where r =( x , y ) is the distance from the vortex centre, λ is the penetration depth and z 0 is the distance from the sample surface to the 2DEG of the Hall cross, the magnetic field profile of a vortex can be closely approximated by the monopole model with the following expression [40] , [41] , [42] : Here, B z ( r ) is the magnetic field perpendicular to the sample surface and Φ is the total flux carried by a vortex. According to ref. 43 , the accuracy of the model can be improved by averaging over an area representative of the Hall probe active area to account for the convolution of the field over the probe. The integration of equation (2) over a square active area of size s divided by the area s 2 gives the following result: where Z = λ + z 0 . For our measurements, a Hall probe with an active area of s 2 =0.4 × 0.4 μm 2 is used. TDGL simulation The TDGL approach (see, for example, ref. 36 ) provides a convenient tool for simulating both dynamic and static properties of superconductors. For a superconductor with pinning centres, which correspond to a local reduction of the mean free path l , the TDGL equation for the order parameter ψ , normalized to 1, can be written as where ϕ and A are the scalar and vector potentials, respectively, and l m is the mean free path outside the pinning centres. The relevant quantities are made dimensionless by expressing length in units of , time in units of πħ /(4 k B T c )≈11.6 τ GL , magnetic field in units of Φ 0 /(4 πξ 2 )= μ 0 H c2 /2 and scalar potential in units of 2 k B T c /( πe ). Here, μ 0 is the vacuum permeability, τ GL is the Ginzburg-Landau time and ξ is the coherence length outside the pinning centres. The vector potential A , for which we choose the gauge ∇ · A =0, can be represented as A = A 0 + A s . Here A 0 denotes the vector potential corresponding to the externally applied magnetic field B 0 , whereas A s describes the magnetic field induced by the currents j , which flow in the superconductor: where κ =λ/ ξ is the Ginzburg-Landau parameter and the current density is expressed in units of with j c , the critical (depairing) current density of a thin wire or film [36] . Integration in equation (5) is performed over the volume of the superconductor. In general, the total current density contains both the superconducting and normal components: j = j s + j n with where σ is the normal-state conductivity, which is taken as σ =1/12 in our units [44] . The distribution of the scalar potential ϕ is determined from the condition which reflects the continuity of currents in the superconductor. Both j n and ϕ vanish when approaching (meta)stable states, which are of our main interest here. We assume that the thickness of the superconductor film is sufficiently small, so that variations of the order parameter magnitude across the sample as well as currents in the this direction are negligible and equation (4) becomes effectively two-dimensional. The equations (4) (5) and (8),  are solved self-consistently following the numerical approach described in ref. 45. How to cite this article: Ge, J.-Y. et al . Bound vortex dipoles generated at pinning centres by Meissner current. Nat. Commun. 6:6573 doi: 10.1038/ncomms7573 (2015).